A genetically female brain is required for a regular reproductive cycle in chicken brain chimeras Sexual differentiation leads to structural and behavioural differences between males and females. Here we investigate the intrinsic sex identity of the brain by constructing chicken chimeras in which the brain primordium is switched between male and female identities before gonadal development. We find that the female chimeras with male brains display delayed sexual maturation and irregular oviposition cycles, although their behaviour, plasma concentrations of sex steroids and luteinizing hormone levels are normal. The male chimeras with female brains show phenotypes similar to typical cocks. In the perinatal period, oestrogen concentrations in the genetically male brain are higher than those in the genetically female brain. Our study demonstrates that male brain cells retain male sex identity and do not differentiate into female cells to drive the normal oestrous cycle, even when situated in the female hormonal milieu. This is clear evidence for a sex-specific feature that develops independent of gonadal steroids. Sexual dimorphism includes biochemical, physiological and morphological differences between males and females, and extends from gonadal differences to differences in other somatic tissues, including the brain. Sexually dimorphic differentiation of the brain leads to the expression of sex-specific behaviour. The molecular mechanisms underlying gonadal development have been studied extensively. Genes located on the Y chromosome, including the SRY gene in mammalian species [1] , [2] , [3] and DMY in some fish [4] , are critical for testis development. In contrast to gonadal development, most evidence suggests that the brain is masculinized during the foetal or neonatal period by the action of androgen hormones secreted from the testes, regardless of the presence of the SRY gene in brain tissue. This causes expression of the male pattern of neural differentiation and behaviour in mammals [5] , [6] . In rodents, androgen secreted from the testes is converted to 17β-oestradiol (E2) by aromatase in the brain, leading to sexual differentiation [7] . Thus, the action of hormonal factors during a critical period of development is thought to be essential for sexual differentiation of the mammalian brain. This theory also applies to Aves, in which the sex chromosomes are Z and W, ZZ being male and ZW being female. The DMRT1 gene on chromosome Z has been shown to be required for testis determination [8] . The DMRT1 gene is not subject to dosage compensation, and the amount produced in females is insufficient to make a testis. Instead, the ovary develops from the gonadal primordium. Recently, Zhao et al. [9] showed that the development of somatic tissues including gonad in the naturally occurring mixed-sex chimeric chicken is a cell-autonomous phenomenon that is independent of hormone effects. From day 6.5 of incubation (ED6.5), the ovaries contain a greater amount of E2 than do the testes; moreover, plasma levels of E2 are higher in females than in males from ED14, whereas gonadal and plasma testosterone (T) levels are comparable in embryos of both sexes [10] , [11] . When genetically male chick embryos were treated with T or E2 before ED13, subsequent male mating behaviour induced by T was not observed [12] . Conversely, genetically female chicks were phenotypically sex-reversed by injection of aromatase inhibitor before ED7; the chicks possessed two testes with mature sperm and exhibited male behaviour [13] . The role of E2 in neural and behavioural development has also been shown in quail (for a review, see ref. [14] 14). Because the activity of 5β-reductase is very high during the embryonic stage in Aves, a considerable amount of T is transformed into an inactive form (5β-dihydrotestosterone); this may protect the male brain from becoming behaviourally demasculinized by E2, which is generated from T [15] . Thus, in Aves, the embryonic ovary is more active than the embryonic testis in producing steroids, and the male brain develops in the absence of E2 (default type), whereas E2 produced and secreted from the embryonic ovary feminizes and/or demasculinizes the brain. On the other hand, there is accumulating evidence suggesting that sexual differentiation of the brain occurs, at least in part, independently of steroid hormones. Midbrain dopamine neurons show sexual dimorphism in rodents, and this is controlled directly by the SRY gene [16] , [17] . In naturally occurring gynandromorphic finches, the neural song circuit in the right hemisphere has a more masculine phenotype than that in the left hemisphere, despite the influence of steroid hormones, which should be identical on both sides [18] . To elucidate the extent to which sexual dimorphism is genetically determined, we used chicken chimeras, which provide a view of sexual differentiation in the brain under natural physiological conditions. Chicken chimeras with grafted brain tissues were viable and healthy although medication was needed to suppress immune rejection from occurring in male chimeras grafted with female brain. In female chimeras with a male brain, the onset of egg laying was delayed and its interval was irregular, but its behaviour, plasma concentrations of sex steroids and luteinizing hormone (LH) were similar to typical hens. In contrast, male chimeras with female brains were equivalent to typical cocks. During the perinatal period, the concentrations of oestrogen was elevated more in the male brain compared with female brain. These results indicate that the genetic differences in the brain tissue, independent of hormonal milieu in blood, is an indispensable prerequisite for sexually dimorphic reproductive function. Construction of chimeras Using a surgical method, we replaced the brain primordium of a chick embryo with another one before development of the gonads [19] , [20] . These brain chimeras were allowed to hatch, and their phenotypes were compared among chimeras and with control cocks (M control) and hens (F control). We successfully obtained and analysed 31 brain chimeras ( Fig. 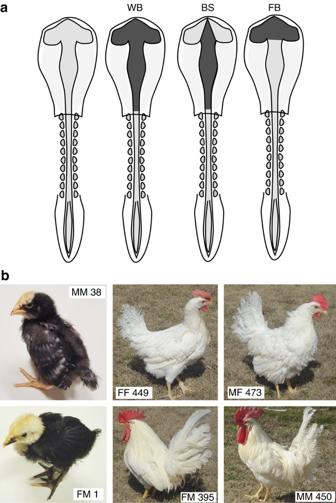Figure 1: Construction of chicken brain chimeras and their appearance. (a) Brain primordium together with mesenchyme and surface ectoderm was exchanged between embryos before development of the gonadal primordium. Three types of grafting (black region in the schema) were performed: WB, BS and FB transplantation. (b) Appearance of the chimeras. MM 38 and FM 1 received FB and BS grafts, respectively, and the yellow pigmentation originated from the grafted tissue (Hypeco chicken) (MM 38 at PD11 and FM 1 at PD17). All other White Leghorn chimeras presented in this panel received a WB graft from White Leghorn chickens. FF 449 chimera at PD731, MF 473 chimera at PD708, FM 395 chimera at PD752 and MM 450 chimera at PD730. FM 395 and MM 450 chimeras were treated daily with Prograf, an immunosuppressive agent, from PD120. This treatment prevented immune rejection in FM 395. 1 and Table 1 ). In the whole brain (WB) chimeras, the WB primordium along with overlaying ectoderm and surrounding mesenchyme extending to the anterior edge of the first somite was grafted; thus, the forebrain (FB), midbrain, isthmus and roughly the rostral half of the hindbrain were of graft origin [21] . The grafted tissue developed normally and incorporated perfectly into the host tissue ( Supplementary Fig. S1 ). To clarify the origin of the pituitary, we used a quail-chick chimera in which quail cells could be traced using a quail-specific antibody, QCPN ( Supplementary Fig. S2 ). In the four chick chimeras with whole quail brain, the percentage of QCPN-positive cells in the pituitary was 85.7±1.7%. On the other hand, in the two quail chimeras with whole chick brain, 4.1% of the cells were QCPN-positive. These results revealed that most of the pituitary was of graft origin. Because the cells of host origin often localized around the blood vessels, at least some of the host cells in the pituitary were endothelial cells. Figure 1: Construction of chicken brain chimeras and their appearance. ( a ) Brain primordium together with mesenchyme and surface ectoderm was exchanged between embryos before development of the gonadal primordium. Three types of grafting (black region in the schema) were performed: WB, BS and FB transplantation. ( b ) Appearance of the chimeras. MM 38 and FM 1 received FB and BS grafts, respectively, and the yellow pigmentation originated from the grafted tissue (Hypeco chicken) (MM 38 at PD11 and FM 1 at PD17). All other White Leghorn chimeras presented in this panel received a WB graft from White Leghorn chickens. FF 449 chimera at PD731, MF 473 chimera at PD708, FM 395 chimera at PD752 and MM 450 chimera at PD730. FM 395 and MM 450 chimeras were treated daily with Prograf, an immunosuppressive agent, from PD120. This treatment prevented immune rejection in FM 395. Full size image Table 1 List of the chimeras. Full size table Chimeras of all types grew up in a healthy state as normal chicks and juvenile chickens until sexual maturity. Male chimeras with male brains (MM chimeras) and with female brains (FM chimeras) were comparable and indistinguishable from normal cocks, and female chimeras with female brains (FF chimeras) and with male brains (MF chimeras) were comparable to normal hens. However, between 122 and 159 days after hatching (PD122–159), we noticed that in the FM chimeras of both Hypeco and White Leghorn origin, the crest and facial skin derived from the grafted tissue became yellowish and swollen. These were observed not only in WB chimeras, but also in FB and brain stem (BS) chimeras of FM combination ( Table 1 ). We observed extensive infiltration of blood cells and tissue injury in the brains of these chimeras ( Supplementary Fig. S3 ). This immune rejection of the grafted tissue was observed in all FM chimeras, but not in other types of chimeras. Because this prevented us from analysing the phenotype of FM chimeras, the FM chimeras that hatched thereafter were treated with the immunosuppressive drug Prograf (tacrolimus hydrate, Astellas, Tokyo, Japan). We first treated control cocks daily with Prograf (0.5 mg per cock per day) for 3 months and confirmed that it did not affect the overall condition of the cocks (data not shown). Starting from PD120, several male WB chimeras and M controls of White Leghorn origin were treated daily with Prograf; this treatment successfully suppressed the rejection of the FM chimeras ( Table 1 , Fig. 1b ). Then, detailed analyses of the WB chimeras of White Leghorn origin were performed. Reproductive characteristics First, we compared the onset of egg laying as an index of sexual maturation in females, between controls and chimeras of White Leghorn origin. Although F controls and FF chimeras both started to lay eggs around PD145 (F, 147.4±2.0, n =17; FF, 142.3±6.1, n =3; n.s., analysis of variance (ANOVA) with Fisher’s protected least significant difference (PLSD)), the onset in MF chimeras was delayed by about 25 days (170.5±4.6, n =4; P <0.05, compared with F and FF, ANOVA with Fisher’s PLSD; Fig. 2a , see also Supplementary Table S1 for P values). When the egg production rate during the first 6 months after the onset was calculated for these birds, F controls and FF chimeras laid similar number of eggs per month (F, 23.5±0.7, n =17; FF, 22.0±2.4, n =3; n.s., ANOVA with Fisher’s PLSD), whereas MF chimeras laid fewer eggs ( Fig. 2b , 8.2±0.8, n =4; P <0.01 compared with F and FF, ANOVA with Fisher’s PLSD). Some birds were kept under a constant light condition and continuously video monitored for 10 days, and the timing of oviposition was checked and its interval was calculated. Mean intervals were 1.03 and 1.08 day for F controls and FF chimeras, respectively, and, as expected, the interval was elevated by 50% for MF chimeras ( Fig. 2c , 1.5±0.1 day). The decrease in frequency of oviposition in MF chimeras was also supported by the data obtained from Hypeco FB chimeras. Two FF chimeras (no. 44 and 48) laid 25.6±1.0 and 28.6±0.8 eggs per month, whereas two MF chimeras (no. 26 and 27) laid 0.8±0.8 and 19.9±1.0 eggs per month. In the ovaries of MF chimeras with WB grafts, large follicles and/or atretic follicles were often found, and hierarchical follicle weight distribution was disturbed ( Fig. 2d and Supplementary Fig. S4 ). To clarify whether these abnormalities could have stemmed from an early developmental defect of the gonad, we histologically compared embryonic gonads of each type of chimera at ED17–19 ( Supplementary Fig. S5 ). We performed in situ hybridization using cRNA probes for aromatase , DMRT1 and Sox9 . Aromatase is known to be expressed by cells in the medullary region of the ovary [22] , and similar expression was observed in FF and MF chimeras. In contrast, expression of DMRT1 (ref. 23 ) and Sox9 (refs 24 , 25 ), markers for the sex cords of the testis, was clearly detected in gonads with a thin-layered cortex and developing sex cords in the medullary region, a typical appearance for a male gonad, in the MM and FM chimeras. These data indicate that early gonadal development was not disturbed. When we housed F controls and FF and MF chimeras with a cock, fertilized eggs were obtained from all birds by natural mating ( Supplementary Fig. S6 ). 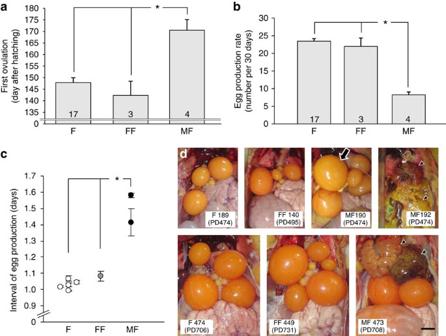Figure 2: MF chimeras showed delayed sexual maturity and a prolonged oestrous cycle. (a) Onset of ovulation was significantly delayed in the MF chimeras as compared with FF chimeras and F controls. (b) MF chimeras produced fewer eggs. (c) The interval of ovulation was prolonged even in the constant light condition in the MF chimeras. Circles indicate the mean values of 10 days observation of individual animals. (d) Development of oocytes in the ovary. At 13–15 months (upper panels), MF chimeras had over-developed follicles (arrow) as well as necrotic follicles (arrowheads). Similarly, at about 24 months (lower panels), necrotic follicles were observed in MF chimeras. Scale bar, 10 mm. *P<0.05, ANOVA with Fisher’s PLSD. The numbers of animals used are indicated in the columns foraandb. Quantified data are presented as mean±s.e.m. Figure 2: MF chimeras showed delayed sexual maturity and a prolonged oestrous cycle. ( a ) Onset of ovulation was significantly delayed in the MF chimeras as compared with FF chimeras and F controls. ( b ) MF chimeras produced fewer eggs. ( c ) The interval of ovulation was prolonged even in the constant light condition in the MF chimeras. Circles indicate the mean values of 10 days observation of individual animals. ( d ) Development of oocytes in the ovary. At 13–15 months (upper panels), MF chimeras had over-developed follicles (arrow) as well as necrotic follicles (arrowheads). Similarly, at about 24 months (lower panels), necrotic follicles were observed in MF chimeras. Scale bar, 10 mm. * P <0.05, ANOVA with Fisher’s PLSD. The numbers of animals used are indicated in the columns for a and b . Quantified data are presented as mean±s.e.m. Full size image Whole-brain FM chimeras started crowing at 2.5–4 months, which was comparable to MM chimeras. When we examined sperm number and activity, the sperm concentration was in the range of 2.1–5.6 × 10 9 ml −1 in all birds, and the indices of sperm motility were similar across the three groups ( Table 2 ). M controls and MM and FM chimeras successfully fertilized eggs when housed with hens ( Supplementary Fig. S7 ). Table 2 Characteristics of the sperm in the semen. Full size table Behavioural analysis The open field and sexual behaviours were analysed ( Supplementary Movies 1–4 and Fig. 3a ). Although hens began to walk around and started pecking or digging after a short period of time, cocks were more cautious and sometimes did not start moving for a few minutes. They did not peck as much, but occasionally they called hens while pecking. We could not detect a difference in the amount of stepping, but pecking frequency was significantly higher in F controls (170.2±22.9 per 10 min, n =16) and FF chimeras (143.5±36.2, n =2) than in M controls (25.1±9.2, n =14) or MM chimeras (10.6±5.7, n =5). Pecking frequency of MF chimeras (188.0±49.3, n =4) did not differ from those of F controls and FF chimeras, but was significantly higher than those of MM and FM chimeras (24.8±5.8, n =2) or M controls. Conversely, the pecking frequency of FM chimeras was comparable to those of M controls and MM chimeras and significantly lower than those of F controls and MF chimeras. These data show that open-field behaviour in brain chimeras is more dependent on the genotype of the body than on that of the brain. 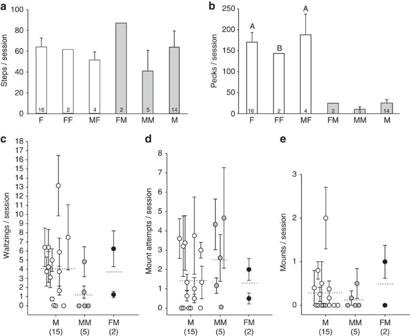Figure 3: Results of behavioural observations. (a,b) In the open-field test, while the number of steps was not significantly different among chimera types (a), F controls and MF chimeras showed significantly more pecks than did FM and MM chimeras, or M controls (b). A,P<0.05 versus FM, MM, M, ANOVA with Fisher’s PLSD; B,P<0.05 versus MM, M, ANOVA with Fisher’s PLSD. (c–e) Male sexual behaviour was compared among M controls, and MM and FM chimeras. There was no significant difference in the frequency of displays of WZ (a), MA (b) or MT (c). WZ and MA were observed in all FM chimeras but never observed in hens. Thus, these behavioural characteristics depended on the sex of the body. The numbers of animals used are indicated in the columns (a,b) or in brackets (c–e). Circles inc–eindicate the mean values obtained from more than three independent observations of each animal and the dashed lines inc–eindicate the mean values for each bird type. Quantified data are presented as mean±s.e.m. Figure 3: Results of behavioural observations. ( a , b ) In the open-field test, while the number of steps was not significantly different among chimera types ( a ), F controls and MF chimeras showed significantly more pecks than did FM and MM chimeras, or M controls ( b ). A, P <0.05 versus FM, MM, M, ANOVA with Fisher’s PLSD; B, P <0.05 versus MM, M, ANOVA with Fisher’s PLSD. ( c – e ) Male sexual behaviour was compared among M controls, and MM and FM chimeras. There was no significant difference in the frequency of displays of WZ ( a ), MA ( b ) or MT ( c ). WZ and MA were observed in all FM chimeras but never observed in hens. Thus, these behavioural characteristics depended on the sex of the body. The numbers of animals used are indicated in the columns ( a , b ) or in brackets ( c – e ). Circles in c – e indicate the mean values obtained from more than three independent observations of each animal and the dashed lines in c – e indicate the mean values for each bird type. Quantified data are presented as mean±s.e.m. Full size image The sexual crouch response to a human hand as an index of sexual receptivity, was tested in F controls and FF and MF chimeras, and was not different among these groups ( Supplementary Movies 5, 6 ). When we tested the M controls and MM and FM chimeras for this response, all of them jumped and none showed a crouching response. For the analysis of male sexual behaviour, we counted the numbers of displays of waltzing (WZ; Supplementary Movies 7, 8 ), mount attempts (MA) and mounts (MT). The frequencies of these responses varied greatly across individuals, but there were no significant differences in these behaviours among M controls (WZ, 4.1±0.9; MA, 1.5±0.4; MT, 0.3±0.1; n =15), MM chimeras (WZ, 1.3±0.9; MA, 2.6±0.9; MT, 0.1±0.1; n =5) and FM chimeras (WZ, 3.7±2.5; MA, 1.3±0.8; MT, 0.5±0.5; n =2; Fig. 3c–e ). Ejaculation was also observed in some birds in each of the three groups, but its frequency was not sufficiently high for a complete analysis. Plasma concentrations of hormones Blood samples were taken from chimeras and controls of White Leghorn origin from 3 to 23 months and plasma levels of sex steroids were analysed. The plasma E2 level remained low in M controls and MM and FM chimeras, whereas it was elevated in F controls and FF and MF chimeras after 4 months of age ( Fig. 4a ). A significant difference was occasionally found in FM chimeras compared with F controls and MF and FF chimeras, but there was no significant difference among FM and MM chimeras and M controls at any age. MF chimeras had significantly higher E2 levels than did FM and MM chimeras and M controls at some ages, but similar levels to those in F controls and FF chimeras at every age. The plasma concentration of T became high in M controls and MM and FM chimeras after 4 months of age, but it remained low in F controls and FF and MF chimeras ( Fig. 4b ). There was no significant difference in plasma T concentration after 4 months among FM and MM chimeras and M controls, or among FF and MF chimeras and F controls. FM chimeras had higher T levels than did F controls after 13 months, and this tendency was observed even earlier. In addition, MF chimeras had lower T levels than did MM chimeras and M controls at some ages. These results show that the plasma levels of sex steroids were similar between chimeras and control birds of the same (body) sex. Chimeras of Hypeco origin yielded similar results except for those that suffered from graft rejection (data not shown). 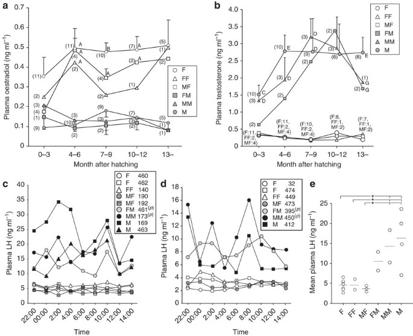Figure 4: Plasma concentrations of sex steroids and the LH secretion pattern. (a) After four months of age, plasma E2 levels were higher in F controls and FF and MF chimeras than in M controls and MM and FM chimeras. (b) In contrast, plasma T levels were higher in M controls and MM and FM chimeras than in F controls and FF and MF chimeras. (c–e) Circadian changes in plasma LH concentrations. At 11–16 (c), or at 21–23 (d) months of age, F controls and FF and MF chimeras showed stable and low levels of LH, whereas M controls and MM and FM chimeras showed fluctuating levels of LH. The mean LH level was higher in M controls and MM and FM chimeras than in F controls and FF and MF chimeras. A,P<0.05 versus FM, MM, M, ANOVA with Fisher’s PLSD; B,P<0.05 versus FM, MM, M, FF, ANOVA with Fisher’s PLSD; C,P<0.05 versus F, FF, FM, MF, ANOVA with Fisher’s PLSD; D,P<0.05 versus F, MF, ANOVA with Fisher’s PLSD; E,P<0.05 versus F, FF, MF, ANOVA with Fisher’s PLSD; G,P<0.05 versus F, ANOVA with Fisher’s PLSD;(P)incandd, Prograf-treated birds. The numbers of animals used are indicated in the brackets foraandb. Fore, circles indicate the mean values obtained during 16 h from individual animals and the dashed lines indicate the mean values for each bird type. *P<0.05, ANOVA with Fisher’s PLSD. Quantified data are presented as mean±s.e.m. Figure 4: Plasma concentrations of sex steroids and the LH secretion pattern. ( a ) After four months of age, plasma E2 levels were higher in F controls and FF and MF chimeras than in M controls and MM and FM chimeras. ( b ) In contrast, plasma T levels were higher in M controls and MM and FM chimeras than in F controls and FF and MF chimeras. ( c – e ) Circadian changes in plasma LH concentrations. At 11–16 ( c ), or at 21–23 ( d ) months of age, F controls and FF and MF chimeras showed stable and low levels of LH, whereas M controls and MM and FM chimeras showed fluctuating levels of LH. The mean LH level was higher in M controls and MM and FM chimeras than in F controls and FF and MF chimeras. A, P <0.05 versus FM, MM, M, ANOVA with Fisher’s PLSD; B, P <0.05 versus FM, MM, M, FF, ANOVA with Fisher’s PLSD; C, P <0.05 versus F, FF, FM, MF, ANOVA with Fisher’s PLSD; D, P <0.05 versus F, MF, ANOVA with Fisher’s PLSD; E, P <0.05 versus F, FF, MF, ANOVA with Fisher’s PLSD; G, P <0.05 versus F, ANOVA with Fisher’s PLSD; (P) in c and d , Prograf-treated birds. The numbers of animals used are indicated in the brackets for a and b . For e , circles indicate the mean values obtained during 16 h from individual animals and the dashed lines indicate the mean values for each bird type. * P <0.05, ANOVA with Fisher’s PLSD. Quantified data are presented as mean±s.e.m. Full size image Because the plasma levels of sex steroids in MF chimeras were similar to those in F controls and FF chimeras, the reduced egg production of MF chimeras could not be attributed to a deficit in sex hormone secretion. Regular egg production, that is ovulation, is supported by periodic changes in LH secretion from the pituitary gland, which is stimulated by gonadotropin-releasing hormone (GnRH). To determine whether this mechanism was affected in the MF chimeras, we performed blood sampling from birds of White Leghorn origin every 2 h and measured plasma LH concentrations at 11–16 months ( Fig. 4c ) or at 21–23 months ( Fig. 4d ). The level of LH was rather low and stable in F controls and FF chimeras ( Fig. 4c ). A surge was observed in some birds (for example, FF 449), but this was not observed in most females during the sampling period (36 h). Therefore, we could not compare the occurrence of surges. However, we did observe stable, low levels of LH in MF chimeras, comparable to those in F controls and FF chimeras. In contrast, the plasma levels of LH in M controls and MM and FM chimeras fluctuated greatly over time, and the levels differed significantly from those in F controls and FF and MF chimeras. Although the range of fluctuation of FM chimeras was somewhat smaller than that in MM chimeras and M controls (with no significant difference), the patterns of fluctuation were similar in the birds of these three groups ( Fig. 4e ). Thus, the pattern of LH secretion into the blood was under the control of the peripheral tissue, probably the gonads. Sexual dimorphism in neurons Sexual dimorphism in the distribution of arginine vasotocin (AVT)- or galanin-expressing neurons in chicken brain has been reported previously [26] , [27] . We examined the distribution of AVT mRNA-expressing neurons in the brains of WB chimeras and controls at 23–25 months and in the brains of FB chimeras at 8–11 months. A sexually dimorphic distribution of AVT neurons was evident in the medial part of the bed nucleus of the stria terminalis (BNSTm). AVT-positive cells were densely packed in this nucleus in M controls and MM chimeras, while these cells were almost absent or only faintly positive cells were observed in F controls and FF chimeras ( Fig. 5 ). In the MF chimeras (no. 281, 26 and 27), the distribution of AVT cells showed the female pattern, whereas the FM chimeras showed the male pattern. The origin of the analysed area was confirmed by the expression of HINTW , a marker specific to the W chromosome. In all MF and FM chimeras, cells of the analysed region were mostly of graft origin, except for some of the blood vessels. Thus, sexually dimorphic expression of AVT in BNSTm cells was dependent on the peripheral tissue, rather than an intrinsic property of the cells. 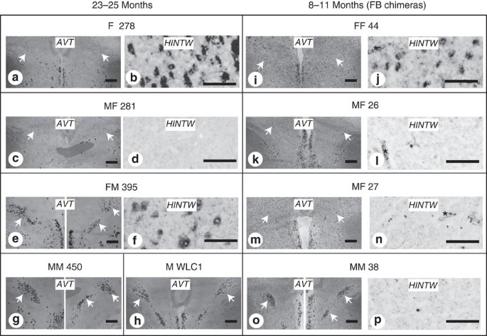Figure 5: Expression ofAVTandHINTWin the BNSTm at 23–25 or at 8–11 months. The chicken brain sections at 23–25 months (a–h) and at 8–11 months (i–p) were processed forin situhybridization. In M controls (h) and MM (g,o) chimeras, densely packed AVT-positive cells were observed in the BNSTm, whereas these cells were not prominent in F controls (a) and FF chimeras (i). FM chimeras (e) showed the male pattern, and MF chimeras (c,k,m) showed the female pattern of AVT-positive cell distribution.HINTWwas expressed in the brains of F controls (b) and FF chimeras (j), but not in the brains of MM chimeras (p), confirming female-specific expression. The female origin of the cells was confirmed by the expression ofHINTWin FM chimeras (f). In the brain sections of MF chimeras, most of the cells wereHINTW-negative (d,l,n). However, endothelial cells of the blood vessels were occasionally positive forHINTWexpression (asterisks inl,n), indicating the invasion of host cells into the grafted tissue, but this was restricted to blood vessel cells. Scale bars ina,c,e,g–i,k,m,o, 500 μm;b,d,f,j,l,n,p, 50 μm. Figure 5: Expression of AVT and HINTW in the BNSTm at 23–25 or at 8–11 months. The chicken brain sections at 23–25 months ( a – h ) and at 8–11 months ( i – p ) were processed for in situ hybridization. In M controls ( h ) and MM ( g , o ) chimeras, densely packed AVT-positive cells were observed in the BNSTm, whereas these cells were not prominent in F controls ( a ) and FF chimeras ( i ). FM chimeras ( e ) showed the male pattern, and MF chimeras ( c , k , m ) showed the female pattern of AVT-positive cell distribution. HINTW was expressed in the brains of F controls ( b ) and FF chimeras ( j ), but not in the brains of MM chimeras ( p ), confirming female-specific expression. The female origin of the cells was confirmed by the expression of HINTW in FM chimeras ( f ). In the brain sections of MF chimeras, most of the cells were HINTW -negative ( d , l , n ). However, endothelial cells of the blood vessels were occasionally positive for HINTW expression (asterisks in l , n ), indicating the invasion of host cells into the grafted tissue, but this was restricted to blood vessel cells. Scale bars in a , c , e , g – i , k , m , o , 500 μm; b , d , f , j , l , n , p , 50 μm. Full size image Neurosteroid concentrations in the brain Accumulating evidence suggests that the brains of songbirds and quail can synthesize steroids de novo [28] , [29] . Because the brain contents of neurosteroids in chicken have not yet been explored, we analysed the brain concentrations of E2, T, 5α- and 5β- dihydrotestosterone in ED21 embryos and adult chickens ( Fig. 6a ). The brains of M controls contained significant greater amounts of E2 than F control brains, both at ED21 ( Fig. 6a ; M, 3.1±0.3, n =5; F, 1.8±0.1, n =5; P <0.05, Student’s t -test) and in adulthood (M, 4.3±0.6, n =5; F, 3.4±0.3, n =5; P <0.05, Student’s t -test). In contrast, brain concentrations of T, 5α- and 5β-dihydrotestosterone in M controls were similar to those in F controls both at ED21 and in adulthood. In MF chimeras at ED21, the brain concentration of E2 was similar to that in MM chimeras (MF, 3.7±0.3, n =6; MM, 3.3±0.1, n =6; n.s. ), but significantly higher than those in FF and FM chimeras (FF, 2.4±0.2, n =7; FM, 2.7±0.1, n =6; P <0.05 compared with FF and FM, ANOVA with Fisher’s PLSD). E2 concentrations in the brains of FM chimeras were comparable to those in the brains of FF chimeras (n.s. ), but significantly lower than those in MF and MM chimeras ( P <0.05, ANOVA with Fisher’s PLSD; Fig. 6b ). These results showed that, in chick, the brain E2 content is higher in males than females, and this sex difference in the perinatal period depends on the sex chromosomal composition in the brain. 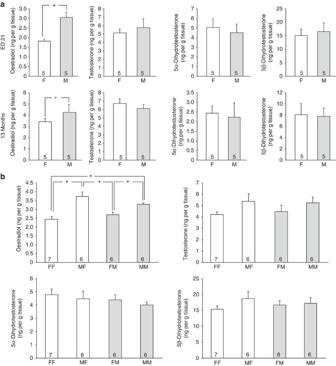Figure 6: Neurosteroid concentrations in the brain. (a) E2 concentrations in the male brain were higher than those in the female brain at ED21 as well as in the adult (13 months). Brain concentrations of T, 5α- and 5β-dihydrotestosterone were similar in males and females at both ages. *P<0.05, Student’st-test. (b) Brain concentrations of E2 in MF chimeras were comparable to those in MM chimeras, but higher than those in FF and FM chimeras. E2 concentrations in FM chimeras were similar to those in FF chimeras but lower than those in MF and MM chimeras. *P<0.05, ANOVA with Fisher’s PLSD. The numbers of animals used are indicated in the columns foraandb. Quantified data are presented as mean±s.e.m. Figure 6: Neurosteroid concentrations in the brain. ( a ) E2 concentrations in the male brain were higher than those in the female brain at ED21 as well as in the adult (13 months). Brain concentrations of T, 5α- and 5β-dihydrotestosterone were similar in males and females at both ages. * P <0.05, Student’s t -test. ( b ) Brain concentrations of E2 in MF chimeras were comparable to those in MM chimeras, but higher than those in FF and FM chimeras. E2 concentrations in FM chimeras were similar to those in FF chimeras but lower than those in MF and MM chimeras. * P <0.05, ANOVA with Fisher’s PLSD. The numbers of animals used are indicated in the columns for a and b . Quantified data are presented as mean±s.e.m. Full size image The immunological rejection of grafted female tissue observed in FM chicken brain chimeras was unexpected, as it had not been reported in allogeneic chicken neural tube chimeras to date [30] . This rejection was strictly sex combination-dependent and, because it started at the time of sexual maturity, it might have been caused by a female-specific antigen coded by a gene(s) on the W chromosome that begins to be expressed at sexual maturity. We did not observe any abnormalities in FM chick chimeras, although a lack of male sexual behaviour has been reported in FM quail chimeras [31] . FM quail chimeras had a lower level of blood T than MM quail chimeras, which could explain this discrepancy. This might be attributed to quail female cells that develop cell autonomously, which could not function as male cells in the quail brain, or a chronic and mild immunological rejection by which functional cells may be gradually eliminated, as in the case of allogeneic forelimb bud grafts [32] . Ovulation in female mammals and birds is exquisitely timed, and is induced by a surge in the secretion of LH. This is ensured by the release of GnRH from hypothalamic neurons into the pituitary portal system. Timed preovulatory activation of GnRH neurons depends mainly on two factors: a rising concentration of E2 during the follicular phase of the oestrous cycle and a circadian timekeeping system. The master circadian pacemaker in mammals is located in the suprachiasmatic nuclei (SCN) of the hypothalamus, and classic experiments have shown that surgical ablation of SCN results in disruption of the oestrous cycle in rats [33] , [34] . Mutations in key circadian rhythm genes such as Clock or Bmal1 in mice affect female reproductive function resulting in an extended and irregular oestrous cycle [35] , [36] . Clock mutant females lack a coordinated LH surge on the day of pro-oestrus, but show normal levels of hypothalamic GnRH, pituitary LH release and plasma E2 and progesterone levels. In MF chick chimeras, blood E2 levels and blood LH fluctuation patterns were normal, despite the extended and irregular oestrous cycle. Thus, the phenotypes of Clock mutant females and chick MF chimeras overlap, suggesting that, in MF chick chimeras, the input of a daily timing signal from the circadian pacemaker centre to GnRH neurons was disrupted. Our results strongly indicate that the input of the circadian signal to GnRH neurons shows sexually dimorphic development, and this occurs independent of the effect of gonadal hormones. In birds, three oscillator systems are known to be involved in the generation of circadian rhythms: the retina, the pineal organ and the SCN [37] , [38] , [39] , [40] , [41] . The circadian pacemaker responsible for determining appropriate ovulation timing as well as the neural circuit that mediates this circadian signalling to GnRH neurons have not yet been elucidated. It will be interesting to investigate the neural basis of this system, which exhibits sex-based differences. Alternatively, because a detailed analysis of the LH surge was not done in this study, defects of the LH surge may be the cause of abnormal ovulation in MF chimeras. GnRH cells originate from the olfactory placode [42] , [43] and this area is included in the grafts of WB but not in those of BS chimeras. Therefore, by comparing BS and WB chimeras, this could be addressed in future work. Our results indicate that sexual dimorphism of the brain E2 concentration is not influenced by gonadal hormone and that the brain may synthesize E2 de novo . Pioneering work has shown the synthesis of E2 from T in the songbird brain [44] . Subsequently, several neurosteroids as well as the enzymes necessary for their production from cholesterol have been found in quail brain [29] , [45] , and there is evidence for de novo synthesis of E2 from cholesterol in songbird brain [28] , [46] . High concentrations of brain E2 may have an organizational effect on the developing male chick brain. The resulting ‘male’ brain, even when situated in the hormonal milieu of the hen, cannot support the regular sexual periodicity seen in hens. Disordered regulation of the ovarian cycle may cause infertility in women. Amenorrhoea, oligo-ovulation and anovulation in women are associated with a number of reproductive disorders including hypothalamic hypogonadism, hyperprolactinemia, polycystic ovarian syndrome and ovarian failure [47] , [48] . In addition, polymorphisms in human clock genes might influence human fertility. A recent genetic analysis of SNPs showed that two clock genes , ARNTL and NPAS2 , are associated with human fertility [49] , although a role for the circadian timing system in human reproduction has not been systematically studied [50] . Elucidation of defects in hypothalamic wiring in MF chimeras may provide new insight into the relationship between the biological clock and fertility. The existence of cell-autonomous development of the brain has been observed in the gynandromorphic finch [18] , and cell-autonomous development of somatic cells has been clearly demonstrated in gynandromorphic chickens [9] . Our present results show a new type of autonomous development of neural cells in birds associated with sexual dimorphism of the brain E2 concentration. Transplantation of the brain primordium Fertilized eggs of Hypeco chickens or White Leghorn ( Gallus gallus domesticus ) were purchased from Shiroyama poultry farm (Kanagawa, Japan) or Akebono farm (Hiroshima, Japan), and were incubated at 37.7 °C. One and half days after beginning incubation (at the 8–10 somite embryonic stage), grafting was performed as described previously [19] . Briefly, after removing 1 ml of egg white, a small portion of egg shell just above the blastoderm was windowed. Under a dissection microscope (MZ7.5, Leica, Germany), the embryonic tissue was visualized by subblastodermal injection of sterile tyrode’s buffer containing 5% black ink (Rotring, Hamburg, Germany). The vitelline membrane above the objective area was removed and the neural tube of the recipient was dissected out using a fine microscalpel. Then the neural tube similarly removed from the donor embryo was grafted isotopically into the recipient. After transplantation, the window of egg shell was sealed with adhesive tape and the egg was kept in the incubator until hatching. As shown in Fig. 1a , three types of replacements were performed: (1) whole-brain (WB) replacement, in which presumptive donor-formed territory was the total brain area, (2) brain stem (BS) replacement, in which presumptive donor-formed territory was the brain stem containing part of the hypothalamus and (3) FB replacement, in which presumptive donor-formed territory was the FB and a part of hypothalamus. To analyse the pituitary origin, fertilized eggs of Japanese quail ( Coturnix coturnix japonica ) were obtained from Toyohashi quail farm (Aichi, Japan). They were incubated under the same conditions as the chicken eggs and used for construction of whole-brain quail/chick chimeras. Animals Chimeras and control chicks that hatched at the early period of this study were raised in the animal facilities of Tokyo Medical and Dental University (Tokyo, Japan), and those that hatched later were hatched and raised in the animal facilities of Tokyo Medical and Dental University or of Kitasato University (Kanagawa, Japan) until 2 or 3 months of age, and then moved to the animal facilities of Hiroshima University (Hiroshima, Japan; Table 1 ). For histological analysis of the brain, for semen analysis and for steroid content measurement, we also used control chickens that were either hatched and grew up in the animal facilities of Hiroshima University, or purchased as adults from a local supplier and maintained and adapted in the animal facilities of Hiroshima University until use. Chicks were housed in groups after hatching, and after 4 months, they were raised in an individual space of a cage unless otherwise specified. They could always see and hear each other. The light cycle was 14 h light/10 h dark unless otherwise specified. Heparinized blood was collected from the wing vein once a month from about 90 days after hatching (PD90). Plasma was prepared by centrifugation and stored at −80 °C until use for E2 and T assays. The number of eggs laid was checked daily and noted. The experimental protocols described in this paper were approved by the Institutional Animal Care and Use Committee of Tokyo Medical and Dental University and for Kitasato University. Open-field test All chickens that reached 4 months of age were tested individually in an open-field test for 10 min. The observation was repeated at least three times over a period of 2 months. The open field consisted of a 1,050 mm (w) × 1,100 mm (d) × 630 mm (h) wire cage with white plastic walls on three sides. Two observers and a video camera (Handycam, Sony, Japan) were settled in front of the open side of the cage. The behaviour was recorded by videotape, and the numbers of steps and pecks were counted. Sexual behaviour For observation of male sexual behaviour, either a control cock or a brain-replaced cock (MM or FM chimera) identified by PCR analysis was placed with two hens for 10 min in the cage used for open-field analysis described above. The behaviour was recorded by videotape and the numbers of WZ, MA, MT and ejaculations were counted. The observation was repeated at least three times on different days over a period of 2 months to 1 year and 7 months, depending on the individual. The combination of a cock and hens was changed occasionally to avoid the preference against a specific hen. It is known that pushing the back of a hen by hand elicits a receptive posture in sexually mature hens [51] . Therefore, for the analysis of female receptive behaviour, we counted the numbers of this response at least three times on different days. E2 and T assay Plasma concentrations of E2 and T were determined using an oestradiol or testosterone enzyme immunoassay (EIA) kit (Cayman Chemical Company, Michigan, USA), respectively. Before analysis, 20 μl of plasma was purified by extraction with diethyl ether and methanol, dried, and suspended in 200 μl of the EIA buffer supplied in the kit. We used 50 μl of this sample for the E2 assay, or this sample was further diluted three times, and 50 μl of this diluted sample was used for the T assay. We followed the assay protocol included in the kit. Determination of the plasma LH concentrations Chickens were individually housed in a room with a constant temperature of 22±2 °C and constant light (24 h light). Chickens were handled during a habituation period of at least 2 weeks. About 0.7 ml of blood was withdrawn from the wing vein of these birds every 2 h for a 36-h period, taking great care to avoid subcutaneous haemorrhage that may prevent further blood collection. After centrifugation, plasma was collected and stored at −80 °C until use. Plasma LH levels were determined by radioimmunoassay (RIA) using a highly purified chicken LH (USDA-cLH-I-3) [52] as the radioligand and standard, and polyclonal rabbit anti-chicken LH serum (USDA-AcLH-5) [52] supplied by the US Department of Agriculture-Agricultural Research Service (USDA-ARS), Biotechnology and Germplasm laboratory (Beltsville, MD). The RIA was performed as described previously [53] , [54] . The antiserum against chicken LH, at a final dilution of 1:50,000, exhibited the ability to specifically bind 23% of the added radioligand in the absence of any unlabelled chicken LH. The sensitivity of the RIA was 0.34±0.07 ng chicken LH per ml assay buffer. The inter-assay and intra-assay coefficients of variation were 7.8% and 6.4%, respectively. Histology of the brain The WB was dissected out from the birds, embedded in the compound and frozen in the powdered dry ice. Six series of 20-μm-thick sections were made with a cryostat (CM1900; Leica Microsystems) and mounted on slide glass, dried and stored at −80 °C until use. One series of sections were fixed with 4% paraformaldehyde overnight and stained with cresyl violet. Other series were fixed with the same solution for 1 h at room temperature and processed for in situ hybridization as described previously [55] . A plasmid containing a fragment of AVT gene was prepared by PCR using chicken brain cDNA as template with primers 5′-agc ctt ccc cga acg cat ag-3′ and 5′-agc act gca gca gac acc a-3′. Examination of the sperm in semen Analysis of sperm concentration and motility to assess quality at ejaculation was done in triplicates by computer-assisted sperm analysis using HTM IVOS Motility Analyzer 8.1 (Hamilton Thorne Research, Beverly, MA, USA) as described previously [56] . Motility is a fraction (%) of spermatozoa population that display movement with a path velocity >10 μm s −1 . Progressive motility is a fraction (%) of spermatozoa population swimming forward with path velocity >25 μm s −1 and straightness >80%. Path velocity is the rate of change of distance along the path, in μm s −1 . Determination of neurosteroid concentrations in the brain Neurosteroid concentrations of E2, T, 5α- and 5β-dihydrotestosterone were determined by gas chromatography/mass spectrometry (GC–MS) (GCMS-QP5000, Shimadzu, Kyoto, Japan) using a CP-Sil 5CB capillary column (Varian, Palo Alto, CA, USA) as described previously [29] , [57] , [58] , [59] . In brief, the WB of birds was homogenized in an aliquot of methanol/H 2 O (75:25 (v/v); 1 ml) on ice. The samples were passed through the C-18 cartridge column, and the neurosteroid fractions were eluted with methanol and dried. Before the measurement of neurosteroids in the brain by GC–MS-selected ion monitoring (SIM), heptafluorobutyrate derivatives of the neurosteroids were prepared by treating the dried samples with heptafluorobutyric anhydride (Wako Pure Chemical, Osaka, Japan) for 30 min at room temperature. For the measurement of neurosteroids, GC–SIM analyses were conducted at m/z 664 for E2, m/z 680 for T, and m/z 486 for 5α- and 5β- dihydrotestosterone. The isoform 5α- and 5β-dihydrotestosterone had different retention times in GC–SIM (5α-dihydrotestosterone at 14.8 min and 5β-dihydrotestosterone at 15.9 min), respectively. The column was maintained at 220 °C for 5 min, and then the temperature was raised to 300 °C at the rate of 5 °C min −1 . Statistical analysis Statistical significance was determined using ANOVA with post hoc Fisher’s PLSD (StatView 5.0; SAS Institute Inc., Cary, NC, USA) for Figs 2a–c , 3a–e , 4a,b,c and 6b . Student’s t -test was used in Fig. 6a . Differences were considered significant for P <0.05. Quantified data are presented as mean±s.e.m., with n as shown in figures or stated in the text. How to cite this article: Maekawa, F. et al. A genetically female brain is required for a regular reproductive cycle in chicken brain chimeras. Nat. Commun. 4:1372 doi: 10.1038/ncomms2372 (2013).